Dearomative di- and trifunctionalization of aryl sulfoxides via [5,5]-rearrangement Aromatic [5,5]-rearrangement can in principle be an ideal protocol to access dearomative compounds. However, the lack of competent [5,5]-rearrangement impedes the advance of the protocol. In this Article, we showcase the power of [5,5]-rearrangement recently developed in our laboratory for constructing an intriguing dearomative sulfonium specie which features versatile and unique reactivities to perform nucleophilic 1,2- and 1,4-addition and cyclization, thus achieving dearomative di- and trifunctionalization of easily accessible aryl sulfoxides. Impressively, the dearomatization products can be readily converted to sulfur-removed cyclohexenones, naphthalenones, bicyclic cyclohexadienones, and multi-substituted benzenes. Mechanistic studies shed light on the key intermediates and the remarkable chemo-, regio- and stereoselectivities of the reactions. Dearomatization represents a powerful strategy for converting readily available arenes to value-added alicyclic compounds [1] , [2] , [3] , [4] , [5] , [6] , [7] , [8] . In contrast with well-established dearomatization protocols such as the Birch reduction, oxidations of phenols, and transition-metal-mediated dearomatizations, etc., the sigmatropic rearrangement-based dearomatizations have not attracted much attention. There have been only sporadic examples of dearomatization via [2,3]- or [3,3]-rearrangement [9] , [10] , [11] , [12] , [13] , [14] , [15] , [16] , which are often limited to ortho, ortho ′-disubstituted benzene derivatives [9] , [10] , [11] , [12] . Li and Lan showcased the potential of benzyne/sulfoxide mediated rearrangement in developing an unique dearomatization reaction [17] , [18] . In theory, [5,5]-rearrangement could enable para -functionalization of benzenes, thus affording para -functionalized alicyclic compounds and broadening the substrate scope. In 1986, Maruyama and Naruta attempted this idea by implementing Claisen-type rearrangement with para -substituted aryl pentadienyl ethers (Fig. 1a ) [19] . In lieu of the expected dearomatization products formed via [5,5]-rearrangement, the reaction generally afforded meta - or ortho -alkylated benzenes. Nevertheless, switching to structurally well-defined substrates like 2,3,4,5-tetrasubstituted aryl pentadienyl ethers, they achieved the first two examples of [5,5]-rearrangement triggered dearomatization. Obviously, the high dependence of specific aryl substituents may severely impede the adoption of the dearomatization protocol. To the best of our knowledge, probably due to the lack of competent [5,5]-rearrangement protocols [19] , [20] , [21] , [22] , [23] , [24] , dearomatization reactions via such rearrangement still remain underexplored. Fig. 1: Background and this work. a Dearomatization via [5,5]-rearrangement by Maruyama and Naruta. b This work: [5,5]-rearrangement-enabled dearomatization of aryl sulfoxides. Full size image During the past few years, a great deal of research effort has been devoted to the development of [3,3]-rearrangements of sulfonium salts derived from aryl sulfoxides [25] , [26] , [27] , [28] , [29] , [30] . The reaction enabled the incorporation of an array of nucleophiles into the ortho -position of aryl sulfoxides while reducing sulfoxides to sulfides, thus providing a powerful synthetic tool for accessing 1,2-disubstituted arenes [31] , [32] , [33] , [34] , [35] , [36] , [37] , [38] , [39] , [40] , [41] , [42] , [43] , [44] , [45] , [46] , [47] , [48] , [49] , [50] , [51] , [52] , [53] , [54] , [55] , [56] , [57] , [58] . Not surprisingly, this type of rearrangements could be coupled with dearomatization processes [44] , [45] , [46] , [59] , [60] , [61] , [62] . For examples, Yorimitsu demonstrated an elegant dearomatization of phenols via their [3,3]-rearrangement with aryl/heteroaryl sulfoxides [44] , [45] , [59] . The [3,3]-rearrangement triggered dearomatization of benzothiophene S -oxides with phenols was also accomplished by Procter [46] , [60] . In addition, we applied the [3,3]-rearrangement to break the aromaticity of ortho,ortho ′-disubstituted aryl sulfoxides and aryl iodanes using difluoro silyl enol ethers and α-stannyl nitriles as rearrangement partner, respectively [61] , [62] . Unlike the well-studied [3,3]-rearrangements of aryl sulfoxides [25] , [26] , [27] , [28] , [29] , [30] , a [5,5]-rearrangement of aryl sulfoxides with allyl nitriles via an “assembly/deprotonation” sequence recently developed in our laboratory allows direct para - in lieu of ortho -C–H alkylation of aryl sulfoxides [63] . The rearrangement is dramatically accelerated by the congestion release of ketenimine moieties embodied in rearrangement precursors, thus the rearrangement could occur at very low temperature (−100 °C) and complete within a few seconds [63] , [64] , [65] , [66] . The effective [5,5]-rearrangement inspired us to quest its capability of unlocking aromaticity of arenes. In this Article, we showcase the potential of the [5,5]-rearrangement for dearomatization of aryl sulfoxides and reveal the versatile reactivities of the rearrangement-enabled dearomatization intermediates (Fig. 1b ). In contrast with the reported stable dearomatization product formed via [5,5]-rearrangement of pentadienyl ethers (Fig. 1a ), the dearomative sulfonium species generated from our [5,5]-rearrangement are unstable at elevated temperature, but allowing for further manipulations at low temperature (−70 °C). The present study demonstrates that the in situ formed intermediate exhibits high electrophilicity and versatile reactivities towards a diverse of nucleophiles and cyclization partners. As a consequence, the protocol allows the installations of two different functionalities into aryl sulfoxides affording value-added alicyclic compounds which can be readily desulfurized to a wide variety of synthetic useful multi-substituted cyclohexenones, naphthalenones and benzenes etc. 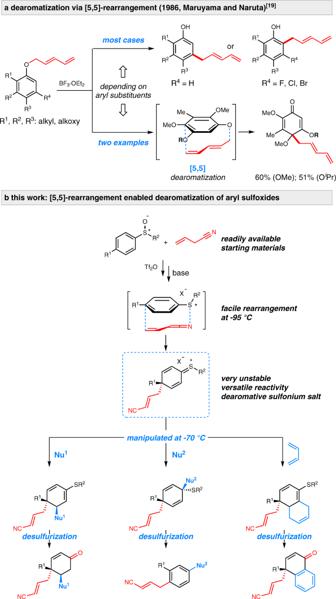Fig. 1: Background and this work. aDearomatization via [5,5]-rearrangement by Maruyama and Naruta.bThis work: [5,5]-rearrangement-enabled dearomatization of aryl sulfoxides. Development of the reaction At the beginning, we examined the [5,5]-rearrangement of para -substituted aryl sulfoxide 1a with allyl nitrile 2a under the conditions we previously developed [63] (Table 1 ). Silyl enol ether 3a was employed as a nucleophile to trap the in situ formed dearomatization species. DABCO previously identified as superior base for deprotonative construction of rearrangement precursor proved unsuitable for the rearrangement of 1a (entry 1). However, when switching to DIPEA, the one-pot three-step reaction afforded desired dual functionalized dearomatizaiton product 4a in modest yield (40% NMR yield). Remarkably, the reaction exclusively produced 1,4-addition product 4a with single diastereomer, exhibiting an excellent regio- and stereoselectivity. The relative configuration of 4a was deduced by single-crystal X-ray analysis of its analog 4l (Fig. 2 ). Among various organic bases (entries 1–6), 4-ethylmorpholine appeared to be optimal, affording 4a in 70% NMR yield (entry 5). Afterwards, the investigation of reaction temperature (T 1 ) and reaction time (t 1 ) revealed that the rearrangement partners assembled at −55 °C for 18 h could increase the yield of 4a to 79% (entries 7–10). Optimization of temperature (T 2 ) and time (t 2 ) for trapping dearomatization species with 3a could not further enhance the efficiency of the reaction (entries 11–14). Comparing with the sequential addition (entry 9), the addition of base and nucleophile in one portion produced nearly the same yield of 4a (entry 15). This result indicated that silyl enol ether 3a could be tolerated in the stage of base promoted deprotonation/rearrangement. For simple operation, the base and nucleophile were added in one portion in the following study unless otherwise noted. It should be noted that the reaction under optimal conditions still furnished a slight amount of undesired ortho -cyanoalkylated product 5 (6% yield). Table 1 Development of the Reaction a Full size table Fig. 2: Dearomative 3,4-dual functionalization of aryl sulfoxides. Reactions were performed under optimal conditions given in Table 1 , entry 15. Base (4-ethylmorpholine) and Nu were added in sequence ( 4u - 4y , 4a′ , 4b′ , 6j and 6k ) or in one portion (others). For cases given below dashed line, sily enol ether 3a or vinyl zinc chloride 3t were used as nucleophile. Unless otherwise noted, only one diastereoisomer was obtained. dr = diastereoisomeric ratio. [b] The absolute configuration of major isomer of 4n is not confirmed. [c] Nu (3.0 equiv) was used. [d] 4-Ethylmorpholine (4.0 equiv) was used. [e] Tf 2 O, −55 °C, 36 h. [f] DIPEA instead of 4-ethylmorpholin was used. [g] Nu, −95 °C, 12 h. [h] 2a (10 equiv) was used. [i] 6k and 6l were contaminated with small amounts of inseparable 1,2-addition products 6k′ and 6l′ with 86/14 rr and 83/17 rr, respectively. [j] In lieu of 6p and 6q , aryl sulfides 7 and 8 were obtained in 40% and 80% yields, respectively. Full size image Scope of the methodology Next, the generality of the dearomative 3,4-dual functionalization reaction was investigated under the optimal conditions (Fig. 2 ). Gratifyingly, a wide variety of nucleophiles including silyl enol ethers ( 4a - 4n ), electron-rich arenes and heteroarenes ( 4o - 4t ), organozinc reagents ( 4u - 4y ) and heteroatom nucleophiles ( 4z- 4b′ ) proved to be suitable for the reaction. As a result, carbonyl groups ( 4a - 4n ), arenes/heteroarenes ( 4o - 4t ), vinyl group ( 4u ), alkynyl groups ( 4v - 4y ), sulfur group ( 4z ), ethoxy group ( 4a′ ) and hydroxyl group ( 4b′ ) were smoothly anchored on the meta -position of aryl sulfoxides. It is impressive that the transformations consisted of three independent steps but still exhibited a high efficiency to afford 3,4-dual functionalized dearomatization products in generally good yields. Furthermore, in all cases, the reaction showcased excellent regio- and stereoselectivity producing single diastereomers. The X-ray diffraction analysis unambiguously demonstrated the relative configuration of 4l . Other products were assigned by analogy to 4l . Interestingly, the feasibility of stereoselective addition was proved by using chiral auxiliary modified silyl enol ether 3n as nucleophile which produced 4n with a modest diastereoselectivity (75/25 dr). It is worthy of noting that the multi-component reaction also demonstrated an excellent functional group (FG) compatibility. A wide range of FGs including aldehyde ( 4f ), arenes/heteroarenes ( 4o - 4t ), vinyl group ( 4u ), alkynyl groups ( 4v - 4y ), and heteroatoms ( 4z - 4b′ ) were all tolerated in the reaction. The excellent FG compatibility can be attributed to the independent and precise control of each step of the reaction and the mild reaction conditions. In addition, the scope of aryl sulfoxides and nitriles was studied under the optimal conditions (Fig. 2 , below the dashed line). 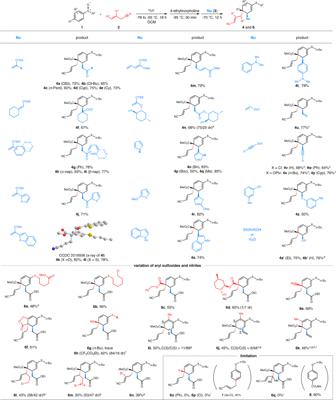Fig. 2: Dearomative 3,4-dual functionalization of aryl sulfoxides. Reactions were performed under optimal conditions given in Table1, entry 15. Base (4-ethylmorpholine) and Nu were added in sequence (4u-4y,4a′,4b′,6jand6k) or in one portion (others). For cases given below dashed line, sily enol ether3aor vinyl zinc chloride3twere used as nucleophile. Unless otherwise noted, only one diastereoisomer was obtained. dr = diastereoisomeric ratio.[b]The absolute configuration of major isomer of4nis not confirmed.[c]Nu (3.0 equiv) was used.[d]4-Ethylmorpholine (4.0 equiv) was used.[e]Tf2O, −55 °C, 36 h.[f]DIPEA instead of 4-ethylmorpholin was used.[g]Nu, −95 °C, 12 h.[h]2a(10 equiv) was used.[i]6kand6lwere contaminated with small amounts of inseparable 1,2-addition products6k′and6l′with 86/14 rr and 83/17 rr, respectively.[j]In lieu of6pand6q, aryl sulfides7and8were obtained in 40% and 80% yields, respectively. In addition to “ n -Bu” group, the substituents on sulfur alkyl group such as ester ( 6a ) and halide ( 6b ) groups could also be well accommodated. The introduction of a chiral auxiliary group to para -ester group failed to induce any stereoselectivity wherein 6d was obtained with 1/1 dr. To our delight, besides para -ester groups, the reaction of para -cyano substituted aryl suloxide afforded a good yield of 6e (69% yield). Remarkably, a structurally appealing bicyclic product 6f was obtained in a good yield (61%). para -Methyl substituted aryl sulfoxide failed to furnish desired 6g . However, switching S-substituent from “ n -Bu” to “CF 2 CO 2 Et” could change the fate of the reaction to afford dearomatization product 6h in a good yield (62%). We speculated that the electron-withdrawing group would increase the electrophilicity of activated sulfoxide and thus enhance the assembly of sulfoxide and allyl nitrile which has been studied previously in our laboratory [55] Meanwhile, we do not believe the “fluoro alkyl” group could exert any special influence on the rearrangement process. The reaction of ortho -methyl substituted aryl sulfoxide gave rise to the formation of regioisomers 6i in 50% yield with 11/89 rr. The use of vinyl zinc reagent as nucleophile slightly increased the regioselectivity affording 6j with 6/94 rr. Impressively, despite steric hinderance, the 1,4-addition of vinyl zinc chloride still proceeded smoothly to give intriguing 3,4,5-densely-substituted 6k albeit accompanied by a small amount of 1,2-addition product (7% yield). Remarkably, in addition to simple allyl nitrile ( 2a ), γ-alkylated allyl nitriles ( 2b and 2c ) and β-bromo-allyl nitrile ( 2d ) were all adopted by the reaction albeit with relatively low yields ( 6l , 43%; 6m , 50% and 6n , 39%) and poor diastereoselectivity ( 6l , 58/42 dr and 6m , 53/47 dr). para -Ph or Cl-phenyl sulfoxides failed to produce any desired products 6o and 6p . Interestingly, dechlorination product 7 was obtained from the reaction of para -Cl phenyl sulfoxide. Probably due to steric hinderance, γ-dialkylated allyl nitrile 2e could not lead to any desired 6q . Instead, aryl sulfide 8 resulted from reduction of sulfoxide was obtained in 80% yield. In contrast with 1,4-addition of silyl enol ether 3a (Fig. 2 ), the use of β-alkylated silyl enol ethers ( 9 ) and aryl amines ( 10 and 11 ) as nucleophile led to a complete regioselectivity switch achieving dearomative 1,4-dual functionalization of aryl sulfoxides (Fig. 3 ). In addition to β-alkyl silyl enol ether 9a , β,β′-dialkyl silyl enol ethers 9b - 9g smoothly afforded 14b - 14g constructing two adjacent quaternary stereocenters. The relative configuration of 14d was unambitiously confirmed by its X-ray structure that was also used for assigning the stereochemistry of other products. Similar to the 1,4-addition pattern shown in Fig. 2 , the reaction proceeding via 1,2-addition also showcased excellent regio- and stereoselectivity. In addition to 1a , meta -chloridephenyl sulfoxide and para -cyanophenyl sulfoxide were also suitable for the reaction albeit furnishing 14h and 14i in modest yields. Impressively, γ-alkylated allyl nitrile 2b could overcome the steric hinderance to afford 14j in a good yield. Furthermore, N -Ms or Ac protected aryl amines 10a , 10c and 10e were found to be competent nucleophiles to access 1,4-dual functionalized products 15a , 15c , and 15e , respectively. However, Ms or Ac protected aliphatic amines 10b and 10d proved unstuiable for the reaction. 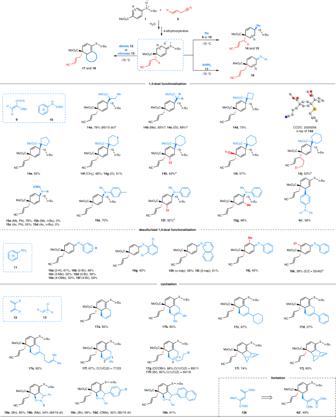Fig. 3: Dearomative 1,4-dual functionalization and dearomative cyclization of aryl sulfoxides. Reactions were performed on 0.5 mmol scale under optimal conditions. 5.0 equiv of dienes and 3.0 equiv of dipoles were used in the reaction. 4-ethylmorpholine and Nu were added in one portion (14a-14c,14j,15a-15gand4c′) or in sequence (others). Unless otherwise noted, only one diastereoisomer was obtained. dr = diastereoisomeric ratio.aTMS-protected enol silyl ethers were used.bNu, −95 °C, 12 h. In contrast with protected aryl aimines, diphenylamine exclusively produced 1,4-addition product 4c′ with C–C bond formation. This result probably reflects a significant impact of steric and electronic effects of nucleophiles on the regioselectivity of the reaction. Fig. 3: Dearomative 1,4-dual functionalization and dearomative cyclization of aryl sulfoxides. Reactions were performed on 0.5 mmol scale under optimal conditions. 5.0 equiv of dienes and 3.0 equiv of dipoles were used in the reaction. 4-ethylmorpholine and Nu were added in one portion ( 14a - 14c , 14j , 15a - 15g and 4c′ ) or in sequence (others). Unless otherwise noted, only one diastereoisomer was obtained. dr = diastereoisomeric ratio. a TMS-protected enol silyl ethers were used. b Nu, −95 °C, 12 h. Full size image Unlike secondary aryl amines, the reaction of primary aryl amines 11 led to quinone imines ( 16 ) with removal of sulfur moieties (Fig. 3 ). Among them, the reaction of unsymmetrical ortho -methyl phenyl sulfoxide proceeded with excellent stereoselectivity to give ( E )-quinone imines ( 16j ). In contrast, meta -chlorophenyl sulfoxide suffered poor stereoselectivity furnishing 16k as a mixture of stereoisomers ( E / Z = 55/45). In addition to 1,4- and 1,2-addition, we further examined the feasibility of cyclization using in situ generated dearomative sulfonium intermediate as shown in Fig. 3 . To our delight, a diverse of cyclization partners were successfully incorporated into aryl sulfoxides via consecutive dearomatization/cyclization process. Dienes 12 were used to trap dearomative sulfonium species via [4 + 2]-cyclization producing various bicyclic compounds 17 . It is remarkable that dienes bearing 2-cyclohexyl ( 12c ), phenyl ( 12d ) groups and alkene tethered alkyl chain ( 12e ) afforded desired products 17c - 17e with excellent regioselectivity. In contrast, small portion of regioisomers were determined when employing 2-methyl, 2-bromoalkyl and 2-carbonate substituted dienes 12f - 12h . Not surprisingly, both cyclopentadiene 12i and cyclohexadiene 12j were well adopted by the reaction. In addition to dienes, nitrones 13 were also found to be competent for trapping the dearomative sulfonium intermediate via [3 + 2]-cyclization leading to structurally appealing hetero-bicyclic compounds 18 . Despite the remarkably high electrophilicity of dearomative sulfonium species, electron-rich diene 12k failed to afford desired bicyclic product 17k wherein 1,4-addition product 4d’ was obtained in a modest yield. Overall, the [5,5]-rearrangement triggered dearomatization followed by either 1,4- and 1,2-addition and cyclization exhibited a remarkable synthetic efficiency of converting readily available aryl sulfoxides to valuable densely-substituted 1,3- and 1,4- cyclohexadienes and bicyclic compounds which can be difficult to make by other known methods. Transformation of products to value-added alicyclic compounds To demonstrate the utility of the reaction, we combined the dearomative 3,4-dual functionalization process with thioenol ether hydrolysis (Fig. 4 ). As a result, the protocol allowed the facile synthesis of a wide variety of cyclohexenones. Impressively, the whole transformation despite consisting of four independent stages still achieved intriguing densely-substituted cyclohexenones in respectful yields (40–73%). It is noteworthy that the final hydrolysis of thioenol ethers had no detrimental effect on dearomatization products. The stereochemistry of rearrangement products and their functional groups such as esters/ketones ( 19a - 19e ), alkene ( 19j ), alkynyl group ( 19k ), and arenes/heteroarenes ( 19f - 19i ) remained intact in the hydrolysis. In addition to excellent regio- and stereoselectivity and remarkable functional group compatibility, the use of readily available starting materials demonstrated the practicality of the protocol for producing polysubstituted cyclohexenones. Fig. 4: One-pot synthesis of cyclohexenones. The reaction was performed on 0.5 mmol scale under optimum conditions. After addition of Nu, the reaction mixture was treated with H 2 SO 4 aq./EtOH at 65 °C for 10 h. In cases of 19a-19k , only one diastereoisomer was obtained. Full size image The unique structures of 1,4-cyclohexediene products 14 and 16 and bicyclic product 17 prompted us to examine their reactivities. As illustrated in eqs 1 and 2 (Fig. 5 ), in presence of AlCl 3 , desulfurization of 14a and 14f was achieved to afford intriguing multi-substituted benzenes 20a and 20f , respectively wherein the ester group shifted from the para to meta -position (eq 1). Basic hydrolysis enabled de-esterification rearomatization of quinone imines 16a , 16i and 16j producing valuable anilines 21a , 21i , and 21j , respectively (eq 2). A consecutive DDQ oxidation and hydrolysis allows for the removal of sulfur moieties of dearomative cyclization products 17 leading to naphthalenones 22a - 22d and cyclohexadienones 22i and 22j (eq 3). As such, the versatile derivatizations of dearomatization products showcases their potential in synthetic applications. Fig. 5: Elaboration of 1,4-cyclohexedienes 14 and 16 and bicyclic products 17. Conditions for eq 1: 14 (0.2 mmol), AlCl 3 (0.5 equiv), DCM, rt, 12 h; Conditions for eq 2: 16 (0.2 mmol), NaOH (10% aq. )/Et 2 O, rt, 12 h; Conditions for eq 3: 17 (0.2 mmol), DDQ (2.0 equiv), THF, 0 °C or rt, 2 h; then H 2 SO 4 aq., rt, 12 h. Full size image The overall mechanism of the reaction To gain insights into the reaction mechanism, density functional theory (DFT) calculations (see SI 8.1 for computational details) were carried out to characterize the detailed pathways for the reaction of 1a with 2a and 3a (Fig. 6a ). 2a has two conformers, namely, s-trans-conformer (s-trans- 2a ) and s-cis conformer (s-cis- 2a ). We first discuss the reaction pathway of s-trans- 2a , colored in black. 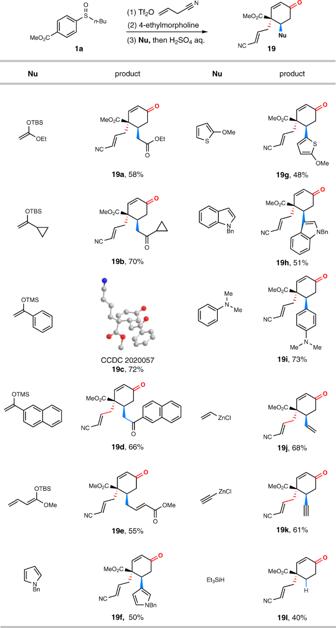Fig. 4: One-pot synthesis of cyclohexenones. The reaction was performed on 0.5 mmol scale under optimum conditions. After addition of Nu, the reaction mixture was treated with H2SO4aq./EtOH at 65 °C for 10 h. In cases of19a-19k, only one diastereoisomer was obtained. To begin with, the activator Tf 2 O activates 1a to enable the formation of the salt IM1 with a mechanism we reported previously [63] . The base 4-ethylmorpholine then deprotonates IM1 via TS1 , followed by OTf - departure, generating the salt IM3 as the rearrangement precursor. By crossing TS3 , dearomative [5,5]-rearrangement takes place to convert IM3 to IM4 . Geometric optimizations to locate a transition state (namely, TS3a ) for [3,3]-rearrangement repeatedly converged to [5,5]-rearrangement transition state TS3 , which, along with the very low [5,5]-rearrangement barrier (0.8 kcal mol −1 , TS3 relative to IM3 ), indicates the strong preference of IM3 to undergo of [5,5]-rearrangement. Finally, the nucleophile 3a intercepts the rearrangement intermediate IM4 via nucleophilic 1,4-addition (see below for more details), affording the product 4a . Overall, the reaction is exergonic by 101.0 kcal mol −1 , with a rate-determining barrier of 6.4 kcal mol −1 ( TS1 relative to IM1 ) for deprotonation. The energetics well explains why the reaction could proceed facilely. Fig. 6: Mechanistic study results. a The overall mechanism of the reaction. b Understanding the formation of 5. c Understanding the regio- and stereoselectivities of the reaction. Full size image The reaction pathway of s-cis- 2a , colored in blue, is similar to that of s-trans- 2a , except for a [3,3]-rearrangement for IM3′ leading to IM4′ and then 5 . Similar to the case IM3 , geometric optimizations to locate a transition state (namely, TS3a′ ) for [5,5]-rearrangement repeatedly converged to [3,3]-rearrangement transition state TS3′ . Thus, IM3 and IM3′ intrinsically prefer [5,5]- and [3,3]-rearrangement, respectively, which we attribute to the longer trans -ketenimine moiety in IM3 than the cis -ketenimine moiety in IM3′ . Comparing the two pathways, the intermediates and the transition states in the blue pathway are all above their counterparts in the black pathway. Notably, TS3′ for [3,3]-rearrangement is 5.7 kcal mol −1 higher than TS3 for [5,5]-rearrangement. Similar to our previous study [63] , we attribute the higher TS3′ than TS3 to the linear ketenimine group which brings up strain in the six-membered [3,3]-rearrangement transition state TS3′ . Understanding the formation of 5 It is interesting that, as the reaction mainly afforded dearomative product 4a , it meantime gave minor rearomatization product 5 (Table 1 ). On the basis of the reaction pathways of s-trans- 2a and s-cis- 2a , we attribute the formation of 5 to the kinetic competition between the two pathways. 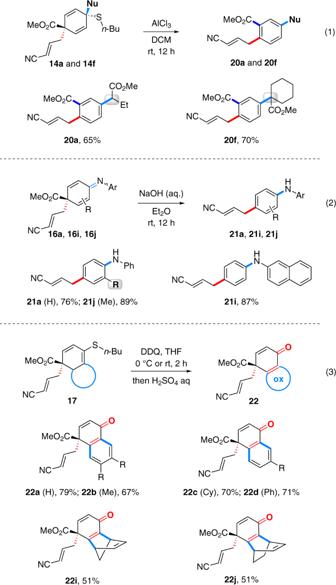Fig. 5: Elaboration of 1,4-cyclohexedienes 14 and 16 and bicyclic products 17. Conditions for eq 1:14(0.2 mmol), AlCl3(0.5 equiv), DCM, rt, 12 h; Conditions for eq 2:16(0.2 mmol), NaOH (10% aq.)/Et2O, rt, 12 h; Conditions for eq 3:17(0.2 mmol), DDQ (2.0 equiv), THF, 0 °C or rt, 2 h; then H2SO4aq., rt, 12 h. Thus, we located the transition states TS5 - TS8 for possible inter-conversions between the two pathways. TS6 and TS7 are 4.1 and 5.7 kcal mol −1 higher than TS2 and TS3 , respectively, thus IM2 or IM3 can be excluded as competition entrances. Because TS5 for the conversion of IM1 to IM1′ is lower than TS1 by 2.5 kcal mol −1 , the two pathways compete at the deprotonation with an energetic difference of 1.7 kcal mol −1 ( TS1′ relative to TS1 ) in favor of the formation of 4a . The energetic difference predicts an 80/1 ratio of IM4 / IM4′ . The formation of IM4′ provides an entry to 5 . Alternatively, IM4 can convert to the more stable 5 via Cope rearrangement via TS8 when 3a was not added. Therefore, two pathways contribute to the formation of 5 , which could be why the experimental yield of 5 (6%) is higher than the predicted yield according to the ratio of IM4 / IM4′ . Note that, because TS8 is much higher than (3a)TS4B by 16.1 kcal mol -1 , the Cope-rearrangement pathway could be excluded when 3a was presented. On the basis of the computed mechanism and the energetics, we reasoned the following: (i) IM1 could be observed in the absence of base, because the reaction can stop at IM1 . IM4 could also be observed in the presence of base but absence of 3a , because IM4 is kinetically stable with a relatively high barrier of 17.0 kcal mol −1 ( TS8 relative to IM4 ). Indeed, at low temperature (−78 °C), we observed both IM1 and IM4 with NMR spectroscopy. It should be noted that the sample of IM4 was pretreated with an acid (CF 3 COOH) prior to NMR measurement since we failed to correct baseline distortions in NMR spectra of the original sample. In addition, IM4 was also detected by ESI-MS. (ii) In the absence of 3a , the reaction could afford 5 through the competitive [3,3]-rearrangement and the feasible Cope rearrangement of IM4 to 5 . To corroborate this, we carried out the control experiment (Fig. 6b ). After in situ generation of IM4 , we stopped the reaction for 1 h at a given temperature (T), and then continued the reaction for 12 hrs by adding 3a at −70 °C. It was observed that as T increases, the yield of 4a decreases, while that of 5 increases. The experimental results agree with (ii), because raising the temperature (T) favors IM4 to undergo irreversible Cope-rearrangement to give 5 during the period of 1 h. Understanding the regio- and stereoselectivities of the reaction In addition to 3a , we further considered the nucleophilic additions of 9d and 11a to IM4 . The pathways for the reactions of 9d and 11a with IM4 to give 14d and 16a , respectively, are detailed in Supplementary Fig. 26 in SI 8. 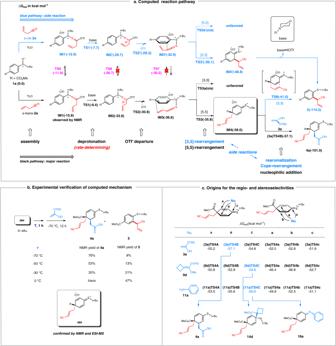Fig. 6: Mechanistic study results. aThe overall mechanism of the reaction.bUnderstanding the formation of 5.cUnderstanding the regio- and stereoselectivities of the reaction. Figure 6c shows the results for the nucleophilic addition step. For each of the three nucleophiles, we considered six possible addition modes and located the corresponding six transition states. Note that addition modes A and B (or a and b) can be differentiated with respect to the S-nBu group and the stereochemistry of para -carbon. Due to the less steric effect of ester group than the cyanoalkyl group lying on the other side, the three nucleophiles all prefer approaching IM4 from its upper face syn to the ester group, in agreement with our observed stereoselectivity of the reaction. The combinations of steric and electronic effects favor 3a to undergo 1,4-addition giving 4a , while 9d and 11a to undergo 1,2- additions to give 14d and 16a , respectively. The energetic results explain our experimentally obtained products. In contrast with well-established dearomatization protocols such as the Birch reduction, sigmatropic rearrangement-based dearomatizations are a less-explored but potentially effective route to saturated compounds. Here, we show a [5,5]-rearrangement-enabled dearomatization of aryl sulfoxides. The key step of the reaction is the in situ formation of an intriguing dearomative sulfonium species via [5,5]-rearrangement of aryl sulfoxides with ally nitrile. This dearomative species is found to be unstable at evaluated temperature but could be manipulated at certain low temperature (−70 °C). Impressively, the intermediate exhibits versatile reactivities towards a wide variety of nucleophiles. As a result, the protocol allows for converting three readily available substrates to a diverse of polysubstiuted 1,3- and 1,4-cyclohexendienes, quinone imines and bicyclic compounds in a regio- and stereoselective manner. Simple elaboration of the dearomatization products produces valuable sulfur-removed cyclohexenones, naphthalenones, bicyclic cyclohexadienones, and multi-substituted benzenes. Mechanistic studies well explain the occurrence of the reaction with excellent chemo-, regio- and stereoselectivities. Further studies of the structurally unique dearomatization products and [5,5]-rearrangement triggered dearomatization reactions are underway. Representative procedure for dearomative di- and trifunctionalization of aryl sulfoxides To a mixture of aryl sulfoxide 1a (120 mg, 0.5 mmol) and allyl nitrile 2a (121 μL, 3.0 equiv) in DCM (3.0 mL) was added Tf 2 O (126 μL, 1.5 equiv) at −78 °C under N 2 amosphere. The mixture was gradually warmed to −55 °C. After stirring for 18 h, the mixture was cooled to −95 °C. To the resulted mixture was added a mixture of 4-ethylmorpholine (157 μL, 2.5 equiv) and silyl enol ether 3a (202 mg, 2.0 equiv) in DCM (2.0 mL) dropwise in 20 min using syringe pump. After stirring for 30 min, the mixture was gradually warmed to −70 °C and further stirred for 12 h. Then the mixture was passed through a short silica gel column and concentrated under vacuum. The obtained residue was further purified by flash chromatography on silica gel affording dearomatization product 4a . For other procedures, see the Supplementary Information .